Ampere-level current density ammonia electrochemical synthesis using CuCo nanosheets simulating nitrite reductase bifunctional nature 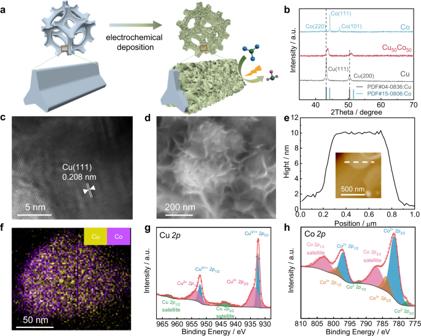Fig. 1: Preparation strategy and characterization of catalysts. aSchematic diagram of CuCo alloy electrodeposition on nickel foam’s surface.bXRD spectra of Cu50Co50, Cu, and Co. HRTEM image (c), SEM image (d), linear topography profiles from AFM images (e), and EDS mapping analysis (f) of Cu50Co50. XPS peaks spectra of Cu 2p(g) and Co 2p(h) of Cu50Co50. The development of electrocatalysts capable of efficient reduction of nitrate (NO 3 − ) to ammonia (NH 3 ) is drawing increasing interest for the sake of low carbon emission and environmental protection. Herein, we present a CuCo bimetallic catalyst able to imitate the bifunctional nature of copper-type nitrite reductase, which could easily remove NO 2 − via the collaboration of two active centers. Indeed, Co acts as an electron/proton donating center, while Cu facilitates NO x − adsorption/association. The bio-inspired CuCo nanosheet electrocatalyst delivers a 100 ± 1% Faradaic efficiency at an ampere-level current density of 1035 mA cm −2 at −0.2 V vs . Reversible Hydrogen Electrode. The NH 3 production rate reaches a high activity of 4.8 mmol cm −2 h −1 (960 mmol g cat −1 h −1 ). A mechanistic study, using electrochemical in situ Fourier transform infrared spectroscopy and shell-isolated nanoparticle enhanced Raman spectroscopy, reveals a strong synergy between Cu and Co, with Co sites promoting the hydrogenation of NO 3 − to NH 3 via adsorbed *H species. The well-modulated coverage of adsorbed *H and *NO 3 led simultaneously to high NH 3 selectivity and yield. Nitrate anions (NO 3 − ), widely present in industrial and agricultural wastewater, pose a real potential threat to human health and ecological balance, especially their incomplete conversion into nitrites (NO 2 − ) which are thought to be cancerogenic by inducing liver damage and methaemoglobinaemia [1] . The conventional biological treatments for NO 3 − removal into nitrogen (N 2 ) gas, involving nitrification and denitrification processes, are energy intensive (~11.7 to 12.5 kWh kg N −1 ) [2] . Actually, the reduction of NO 3 − into NH 3 has become of great interest from an industrial point of view since NH 3 is a highly important industrial chemical for the synthesis of pharmaceuticals, fertilizers, dyes, plastic, etc. [3] , and is also considered for hydrogen storage/release as a carbon-free hydrogen carrier [4] . To date, the industrial synthesis of NH 3 relies heavily on the non-sustainable and eco-unfriendly Haber–Bosch route, which requires harsh conditions i.e., high temperature (400–600 °C) and high pressure (200–350 atm), and heavily relies on fossil energy [3] . The total amount of CO 2 produced during the Haber–Bosch process accounts for roughly 1.2% of the global annual CO 2 emissions, more than any other industrial chemicals synthesis [5] . Electrocatalytic reduction of NO 3 − into NH 3 , powered by green energy, has drawn increasing attention and is considered as a sustainable complementary process to the Haber–Bosch process [2] , [6] , [7] , since this technology can simultaneously meet the 21st session of the Conference of the Parties (COP) two-degree scenario (2DS) target for NH 3 and protect the environment from the eutrophic water pollution. The rational design of novel electrocatalysts with both high activity and selectivity is crucial for reducing NO 3 − (NO 3 − RR) and achieving large-scale applications, and satisfying high industrial demands. Since Nature has developed sophisticated and efficient machinery such as enzymes [8] , [9] , it is interesting to design catalysts by studying the mechanism of enzymatic reduction. Indeed, biocatalytic reduction of NO 3 − to NH 3 widely exists inside many microorganisms, where NO 3 − ions are firstly reduced into NO 2 − by NO 3 − reductases that accept electrons from quinone [10] . The generated NO 2 − is further converted to NH 3 by nitrite reductases (NIRs) using quinone as electron donors. Among various NIRs, the Cu-type NIRs (Cu-NIRs) found in Rhizobium is one of the most important enzymes for N 2 fixation. Cu-NIRs are trimeric proteins composed of 3 identical subunits, and each monomer has two types of Cu atomic active centers, acting as electron-donating centers (T1Cu) and catalytic centers (T2Cu), respectively [10] . The reported mechanism proposes that *NO 2 − (where * denotes an adsorbed specie) is bound to the T2Cu in a bidentate form via two oxygen atoms. Due to the electrons transfer from T1Cu to T2Cu, the T2Cu oxidation state decreases from (II) to (I), facilitating *NO 2 − association with T2Cu in a bridging nitro binding form. Meanwhile, the aspartate acid besides the T2Cu provides proton to one oxygen and extends the N-O bond length, leading to the breaking of the N-O bond [11] . According to the mechanism of NO 2 − reduction on T2Cu and T1Cu, it can be speculated that moderate affinity with NO 3 − , protons availability and electrons provision are the key factors for the high efficiency in NO 3 − RR to NH 3 . Jimmy C. Yu et al. 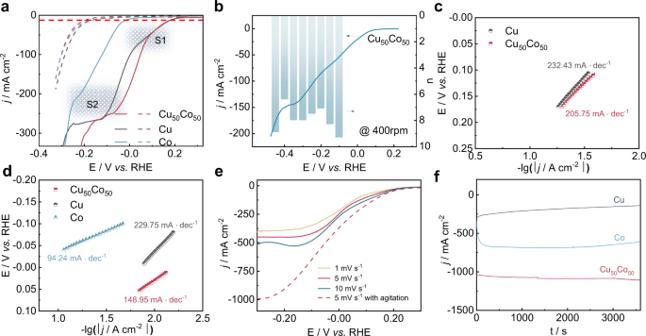Fig. 2: Electrochemical responses of Cu50Co50, pure Cu, and pure Co catalysts. aj-Ecurve (80% iRcorrected) over Cu50Co50, pure Cu, and pure Co modified Ni foams (catalysts loading was 5 mg cm−2) in 1 M KOH solution containing 100 mM KNO3(solid lines) or in the absence of KNO3(dotted line) at a scan rate of 1 mV s−1(the red dash line presenting thejof 10 mA cm−2, the shading S1 and S2 presenting the peak around 0.2 to 0.05 V and 0.05 to −0.15 V, respectively).bj-Ecurve (80% iRcorrected) at 400 rpm and electron transfer numbers at different potentials calculated by the K–L equation for Cu50Co50on RDE in 100 mM KNO3+ 1 M KOH electrolyte at a scan rate of 10 mV s−1(catalysts loading was 0.25 mg cm−2). Tafel slopes in the potential range of peak S1 (c) S2 (d). ej-Ecurves over Cu50Co50modified Ni foam in 1 M KOH solution containing 100 mM KNO3at different scan rates without agitation (solid line) and at a scan rate of 5 mV s−1with agitation (catalysts loading was 5 mg cm−2).fTime-dependent current density curves over Cu50Co50, Cu, Co modified Ni foam at −0.2 V with a magnetic stirring speed of 1000 rpm (catalysts loading was 5 mg cm−2). [12] proved that hydrogen adsorption (*H), with moderate adsorption energy on catalysts, can behave as an important reactive species for the hydrogenation of NO x intermediates to NH 3 whilst suppressing the hydrogen evolution reaction (HER) competition. Matthew J. Liu et al. [13] also found that the NO 3 − RR activity and product selectivity highly depended on the *H coverage on the titanium surface at different potentials with the increase of NO 3 − RR overpotential. Very recently, Schuhmann and his colleagues [14] reported a tandem mechanism for PO 4 3− -modified CuCo binary metal sulfides. They proposed that NO 2 − intermediates were preferentially formed on Cu-based phases followed by splitting over nearby Co-based phases; however, the role of *H during NO 3 − RR was unclear and the effect of the electronic structure of alloyed catalysts on the adsorption of reaction intermediates lacked further discussions in the proposed mechanism [14] . In this study, inspired by the bifunctional nature of the Cu-NIRs, we prepared CuCo alloy nanosheets via a one-step electrodeposition route. The CuCo alloy could well mimic the behavior of the two catalytic centers in Cu-NIRs. The Co species could efficiently provide the electrons and generate the hydrogen protons to the nearby Cu species with high adsorption of NO 3 − and its derivatives. The as-prepared CuCo nanosheet exhibited superior catalytic performances, as (1) the lowest η of 290 mV for ammonia production (at 0.4 V vs. reversible hydrogen electrode (RHE), all electrode potentials mentioned below were provided with respect to RHE unless specially stated); (2) an ampere-level current density of 1035 mA cm −2 with a 100% Faradaic efficiency for NH 3 generation at an overpotential of 890 mV, and a corresponding \({{{{{\rm{Yield}}}}}}_{{{{{{\rm{NH}}}}}}_{3}}\) of 4.8 mmol cm −2 h −1 ; (3) a wide potential window (300 mV, from −0.1 to −0.4 V) for NH 3 generation with >90% Faradaic efficiency (FE), which is one of the most advanced catalysts for NO 3 − RR so far. Electrochemical in situ Fourier transform infrared spectroscopy (FTIR) and in situ shell-isolated nanoparticle enhanced Raman spectroscopy (SHINERS) associated with density functional theory (DFT) calculations were conducted to clarify the pathways and mechanisms of NO 3 − RR, with the aim to contribute to subsequent catalyst optimization and scaling up. Preparation and characterization of CuCo bimetallic electrocatalysts CuCo bimetallic materials were synthesized by co-electrodeposition of Cu and Co on Ni foams’ surfaces (Fig. 1a and Method section). Ni foam is widely used as a supporting substrate for nanostructured electrocatalysts due to its smooth surface and good conductivity, benefiting the electrodeposition by an efficient electron transfer [15] , [16] , [17] . Meanwhile, Ni was proved as a relatively inert material for NO 3 − RR [18] , [19] , without affecting the CuCo catalysts’ performance. The Cu/Co molar ratio was determined using an inductively coupled plasma-optical emission spectrometer (ICP-OES) (Supplementary Table S1 ). The catalyst with a Cu/Co molar ratio of ca . 50/50 was named Cu 50 Co 50 and was considered as a reference in this study. The alloying of Cu and Co in Cu 50 Co 50 was confirmed by X-ray diffraction (XRD) and high-resolution transmission electron microscopy (HRTEM). Indeed, in the diffractogram (Fig. 1b and Supplementary Fig. S1 ) shifts in the Cu (111) and Cu (200) diffraction peaks toward higher degrees were observed after the addition of Co to Cu, which were attributed to the shrinkage of the lattice spacing caused by the partial alloying of Co atom with a smaller diameter compared to Cu atom [20] . Furthermore, the lattice spacing of the Cu (111) plane contracted to 0.208 nm after alloying Cu with Co (Fig. 1c ), when it was 0.212 nm for the Cu (111) plane for the pure Cu catalyst (Supplementary Fig. S2a ) [15] . Scanning electron microscopy (SEM) was applied to examine the morphologies of Cu, Co and Cu x Co y catalysts and showed micro-pines structure for all the catalysts (Supplementary Fig. S3a–j ). At the nanoscale level, small bump structures on the surface of the micro-pines were observed on pure Cu (Supplementary Fig. S3a, b ). After the incorporation of Co, a nanosheet structure emerged on the micro-pine’s surface of the Cu 50 Co 50 catalyst (Fig. 1d and Supplementary Fig. S3e, f), very similar to the structure of pure Co (Supplementary Fig. S3i, j ). The thickness of the Cu 50 Co 50 nanosheet was evaluated by atomic force microscopy (AFM) and was around 10 nm (Fig. 1e ). Besides, the EDS mapping analysis disclosed an even distribution of Cu and Co in Cu 50 Co 50 (Fig. 1f ). Fig. 1: Preparation strategy and characterization of catalysts. a Schematic diagram of CuCo alloy electrodeposition on nickel foam’s surface. b XRD spectra of Cu 50 Co 50 , Cu, and Co. HRTEM image ( c ), SEM image ( d ), linear topography profiles from AFM images ( e ), and EDS mapping analysis ( f ) of Cu 50 Co 50 . XPS peaks spectra of Cu 2 p ( g ) and Co 2 p ( h ) of Cu 50 Co 50 . Full size image The electronic properties of the Cu 50 Co 50 nanosheet were explored by X-ray photoelectron spectroscopy (XPS). Cu 2+ 2 p peaks were observed in the high-resolution Cu 2 p spectra (Fig. 1g ), and was due to the partial oxidation of the alloy’s surface exposed to air, and the same observation was made for Co (Fig. 1h ). The decrease of the Cu 2 p binding energy, compared with pure Cu (Supplementary Fig. S4a ) and the notable increase of the Co 2 p binding energy, compared with pure Co (Supplementary Fig. S4b ), revealed a redistribution of the electrons between Cu and Co after their alloying [21] , leading to the movement of the d band towards the Fermi level [22] comparing with the pure Cu catalyst. X-ray absorption spectroscopy (XAS) analysis was also performed to check the redistribution of electrons between Cu and Co. Extended X-ray absorption fine structure (XANES) spectra depicted a negative shift of the absorption edge position for the Cu K-edge after interacting with Co (indicated by the red arrow in the inset) (Supplementary Fig. S5 ), illustrating the electron density transfer from Co to Cu [23] . In addition, according to the Bader charge analysis (Supplementary Fig. S6 ), compared with monometallic Cu and Co, a charge redistribution on CuCo(111) was observed, where the Cu center displayed a higher electrons density compared to the Co center (Supplementary Fig. S7 ) [24] . The correlation between electrons redistribution within Cu and Co and the adsorption energy of *H, *NO 3 and the *NO x intermediates [25] are discussed further in the mechanistic study section. Electrochemical activity and kinetics of NO 3 − RR NO 3 − RR was first investigated by linear sweep voltammetry (LSV) at a low scan rate of 1 mV s −1 on all the prepared electrocatalysts. The reduction of NO x species contributed mainly to the current density (solid curve), indicating a high catalytic activity toward NO 3 − RR for all the catalysts (Fig. 2a ). The substrate of Ni foam was inactive for NO 3 − RR compared with the electrodeposited catalysts (Supplementary Figs. S8 , S9 ). The overpotential η at 10 mA cm −2 (denoted \({\eta }_{{@{{{{{\rm{10mA}}}}}}{{{{{\rm{cm}}}}}}}^{-2}}\) , η = E o – E , where E is the potential with a current density of 10 mA cm -2 , E o = 0.69 V), where NO 3 − RR is under kinetic control, was used as a criterion to compare the catalysts’ activity. Cu 50 Co 50 and Cu exhibited a lower energy barrier for NO 3 − RR, with \({\eta }_{{@{{{{{\rm{10mA}}}}}}{{{{{\rm{cm}}}}}}}^{-2}}\) of 498 and 503 mV, respectively, compared to Co, that displayed a \({\eta }_{{@{{{{{\rm{10mA}}}}}}{{{{{\rm{cm}}}}}}}^{-2}}\) of 690 mV. In fact, two reduction current peaks (peak S1 and S2) were observed in the curves of Cu and Cu 50 Co 50 . At the initial stage of the reaction, Cu and Cu 50 Co 50 seemed to display a similar behavior toward NO 3 − RR, suggesting the important role of Cu at this stage. According to previous studies [26] , [27] , the peak S1 near 0.08 V was assigned to *NO 3 − (adsorbed NO 3 − ) reduction into *NO 2 − (1) following a 2-electrons transfer process, while the peak S2 was allocated to the *NO 2 − reduction into *NH 3 (2) following a 6-electrons transfer process. In the peak S2 region, Cu 50 Co 50 displayed a positive potential shift of 67 mV, compared to Cu, suggesting a significant synergy between Co and Cu and a drop of the barrier energy of *NO 2 − reduction to *NH 3 , as the applied potential increases. *NO_3^-+2e^-+H_2O→*NO_2^-+2OH^-
 (1) 
    *NO_2^-+6e^-+5H_2O→*NH_3+7OH^-
 (2) Fig. 2: Electrochemical responses of Cu 50 Co 50 , pure Cu, and pure Co catalysts. a j - E curve (80% i R corrected) over Cu 50 Co 50 , pure Cu, and pure Co modified Ni foams (catalysts loading was 5 mg cm −2 ) in 1 M KOH solution containing 100 mM KNO 3 (solid lines) or in the absence of KNO 3 (dotted line) at a scan rate of 1 mV s −1 (the red dash line presenting the j of 10 mA cm −2 , the shading S1 and S2 presenting the peak around 0.2 to 0.05 V and 0.05 to −0.15 V, respectively). b j - E curve (80% i R corrected) at 400 rpm and electron transfer numbers at different potentials calculated by the K–L equation for Cu 50 Co 50 on RDE in 100 mM KNO 3 + 1 M KOH electrolyte at a scan rate of 10 mV s −1 (catalysts loading was 0.25 mg cm −2 ). Tafel slopes in the potential range of peak S1 ( c ) S2 ( d ) . e j - E curves over Cu 50 Co 50 modified Ni foam in 1 M KOH solution containing 100 mM KNO 3 at different scan rates without agitation (solid line) and at a scan rate of 5 mV s −1 with agitation (catalysts loading was 5 mg cm −2 ). f Time-dependent current density curves over Cu 50 Co 50 , Cu, Co modified Ni foam at −0.2 V with a magnetic stirring speed of 1000 rpm (catalysts loading was 5 mg cm −2 ). Full size image In the aim to investigate the reaction routes for all the catalysts, the number of electrons transferred (n) during the NO 3 − reduction reaction was estimated from the slope of the Koutecký–Levich (K–L) plots (Supplementary Fig. S10 ). For the Cu catalyst (Supplementary Fig. S11a ), n was 2 at −0.1 V and a quasi-first-order reaction relationship between j and the NO 3 − concentration was obtained (Supplementary Fig. S12 ), validating the rate-determinate step (RDS) as the reduction route described by Eq. ( 1 ). The n value increased to 6 at −0.25 V, validating the reduction route described in Eq. ( 2 ). In comparison, a direct 8-electrons transfer process was observed on Cu 50 Co 50 in the potential region between the peaks S1 and S2 (Fig. 2b ), revealing a strong alloying effect promoting simultaneously both routes. Though an 8-electrons transfer process also occurred on the pure Co catalyst at a far less negative potential of ca . −0.45 V (Supplementary Fig. S11b ), i.e., at a higher barrier energy. In the potential region of peak S1, the Tafel slopes derived from the j - E curves (Fig. 2c ), for Cu 50 Co 50 was 205.75 mV decade −1 , which was slightly lower than Cu (232.43 mV decades −1 ), indicating that the addition of Co could promote the electrons transfer over the catalyst/electrolyte interface during *NO 3 − reduction to *NO 2 − . This result was supported by EIS data (Supplementary Fig. S13 ), demonstrating a smaller charge-transfer resistance on Cu 50 Co 50 compared to Cu (3.51 vs. 3.81 Ω). The Co catalyst had minor electrocatalytic activity for NO 3 − reduction at this relatively positive working potential, so its Tafel slop in this potential region was not determined. In the potential region of peak S2, the Tafel slope (Fig. 2d ) of Cu 50 Co 50 (148.95 mV decades −1 ) was significantly lower than Cu (229.75 mV decades −1 ); this was explained by an electron redistribution between Cu and Co over Cu 50 Co 50 and was emphasized in the characterization section. The Co catalyst displayed the lowest Tafel slope value of 94.24 mV decades −1 , but at a more negative potential, i.e., 95 mV shift, than Cu 50 Co 50 . This latter result suggested that after crossing a high energy barrier, Co displayed better kinetics’ performances toward the NO 3 − RR for NH 3 production compared to the Cu-based catalysts. Alloying Co to Cu implemented a faster electron transfer rate and improved kinetics’ performances toward the NO 3 − RR. In addition to being affected by the properties of the catalysts, the NO 3 − RR was also diffusion-controlled (Fig. 2e ). To further evaluate the NO 3 − RR activity of the catalysts under steady-state conditions, potentiostatic electrolytic reduction of NO 3 − in a homemade H-type electrolytic cell (Supplementary Fig. S14 ) was carried out by electrodepositing the catalysts on Ni foams’ surfaces. A magnetic stirring rate of 1000 rpm was used to minimize the effect of diffusion and fresh electrolyte solution was constantly supplemented to maintain a constant NO 3 − ion concentration. In these conditions, the current densities obtained on the Cu 50 Co 50 catalyst reached an Ampere level at −0.2 V vs. RHE (Fig. 2f ). NH 3 and NO 2 − were quantitatively detected by the Nessler Reagent method and ion chromatography, respectively (Supplementary Fig. S15 ) [28] , [29] . The gas products were analyzed during the reaction by gas chromatography and online electrochemical mass spectrometry (OEMS) [30] . There was no N 2 production detected and the amount of the stripped NH 3 in this work was negligible. (Supplementary Fig. S16 ) In order to figure out the effect of Co content on the NO 3 − RR activity, CuCo bimetallic catalysts with different Cu/Co ratios were prepared, i.e., Cu 65 Co 35 and Cu 15 Co 85 . As shown in Fig. 3a , when a potential of 0 V was applied, the Faraday efficiency of NH 3 ( \({{{{{\rm{FE}}}}}}_{{{{{{\rm{NH}}}}}}_{3}}\) ) and NO 2 − ( \({{{{{\rm{FE}}}}}}_{{{{{{\rm{NO}}}}}}_{2}^{-}}\) ) on pure Cu were 32% and 60%, respectively. The corresponding molar ratio of NO 2 − to NH 3 was seven times higher (Fig. 3c ), suggesting an accumulation of NO 2 − due to the low kinetic of *NO 2 − hydrogenation to *NH 3 on the Cu surface. With the addition of Co to Cu, both the \({{{{{\rm{FE}}}}}}_{{{{{{\rm{NH}}}}}}_{3}}\) and the geometrically normalized current density of NH 3 production ( \({j}_{{{{{{\rm{NH}}}}}}_{3}}\) ) increased significantly (Fig. 3 a, b ). A volcano shape was observed and the highest \({j}_{{{NH}}_{3}}\) was obtained on Cu 50 Co 50 (i.e., 347 mA cm −2 \({j}_{{{{{{\rm{NH}}}}}}_{3}}\) and 88% \({{{{{\rm{FE}}}}}}_{{{{{{\rm{NH}}}}}}_{3}}\) ), and was ten times higher than monometallic Cu (i.e., 34 mA cm −2 and 32% \({{{{{\rm{FE}}}}}}_{{{{{{\rm{NH}}}}}}_{3}}\) ), and nearly 17 times higher than monometallic Co catalyst (i.e., 21 mA cm −2 and 84% \({{{{{\rm{FE}}}}}}_{{{{{{\rm{NH}}}}}}_{3}}\) ). Furthermore, the molar ratio of NO 2 − to NH 3 exhibited a dramatic drop from 7 to 0.6 as the Co content was raised from 0 to 100% (Fig. 3c ). This observation suggested that the incorporation of Co enhanced further the *NO 2 − hydrogenation into NH 3 . Moreover, when the ratio of Co was increased by over 50%, the \({{{{{\rm{FE}}}}}}_{{{{{{\rm{NH}}}}}}_{3}}\) was remained constant, but the \({{{{{\rm{j}}}}}}_{{{{{{\rm{NH}}}}}}_{3}}\) declined dramatically, indicating that a moderate Cu/Co ratio was important to maintain high catalytic performance for NH 3 production. The electrochemically active surface area (ECSA) was also measured (Supplementary Figs. S17f , S18b ), and all the catalysts had comparable ECSA. The maximum ECSA normalized current density for NH 3 production ( \({j}_{{{{{{\rm{NH}}}}}}_{3}({{{{\rm{ECSA}}}}})}\) ) was obtained on Cu 50 Co 50 (Supplementary Fig. S19 ), indicating that this catalyst had the highest intrinsic activity for NH 3 production. Fig. 3: Electrochemical performance of catalysts. \({{{\mbox{FE}}}}_{{{{\mbox{NH}}}}_{3}}\) and \({{{\mbox{FE}}}}_{{{{\mbox{NO}}}}_{2}^{-}}\) of NO 3 − RR ( a ), bias-current density and products yield for NH 3 ( b ), and the ratio of NO 2 − to NH 3 generated ( c ) for different Cu/Co ratio at 0 V in 100 mM KNO 3 + 1 M KOH electrolyte (catalysts loading was 5 mg cm −2 ). \({{{\mbox{FE}}}}_{{{{\mbox{NH}}}}_{3}}\) ( d ) and NH 3 product yield ( e ) at different electrode potentials on Cu 50 Co 50 , pure Cu and pure Co catalysts modified Ni foam (catalysts loading was 5 mg cm −2 ). Comparison of the electrocatalytic NO 3 - RR performances of Cu 50 Co 50 modified Ni foam with other extensively reported electrocatalysts ( f ). \({{{\mbox{FE}}}}_{{{{\mbox{NH}}}}_{3}}\) and \({{{\mbox{Yield}}}}_{{{\mbox{mass}}}-{{{\mbox{NH}}}}_{3}}\) on Cu 50 Co 50 /Ni foam under the applied potential of −0.2 V during 10 periods of 1 h electrocatalytic NO 3 - RR ( g ) (catalysts loading was 5 mg cm −2 ). The time-dependent concentration of NO 3 − , NO 2 − and NH 3 and corresponding FE over Cu 50 Co 50 modified Ni foam at −0.1 V ( h ) (catalysts loading was 5 mg cm −2 ). Error bars represent the standard deviations calculated from three independent measurements. Full size image To clarify the possible 14 N pollution, the electrolysis in the electrolyte free of NO 3 − ions was performed and little NH 3 was produced (Supplementary Fig. S20 ). \({j}_{{{{{{\rm{NH}}}}}}_{3}}\) in the solution with NO 3 − ions was over 150-fold higher than that in the electrolyte free of NO 3 − . The content of 14 NH 4 + was also analyzed by 1 H NMR test [29] , [31] and was ca . 4.62 mmol cm −2 h −1 . The obtained results were close to the one from the spectrophotometric analysis (4.75 mmol cm −2 h −1 ) (Supplementary Fig. S21d ), and confirmed the reliability of the quantification methods used in this work. The typical two peaks of 15 NH 4 + after the electrolysis of 15 NO 3 − also suggested that the NH 3 product indeed came from the electrocatalytic reduction of NO 3 − (Supplementary Fig. S21e ). It is known that the applied potential influences the products’ selectivity [13] , so we investigated the effect of the applied potential toward the NO 3 − RR (Fig. 3d, e and Supplementary Fig. S22 ). The \({{{{{\rm{FE}}}}}}_{{{{{{\rm{NH}}}}}}_{3}}\) was about 51% at a η of 290 mV (at 0.4 V) on Cu 50 Co 50 . The η was comparatively much lower than that of the state-of-the-art catalysts reported in the literature (Fig. 3f and Supplementary Table S2 ). 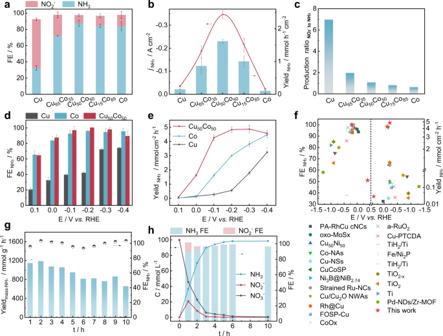Fig. 3: Electrochemical performance of catalysts. \({{{\mbox{FE}}}}_{{{{\mbox{NH}}}}_{3}}\)and\({{{\mbox{FE}}}}_{{{{\mbox{NO}}}}_{2}^{-}}\)of NO3−RR (a), bias-current density and products yield for NH3(b), and the ratio of NO2−to NH3generated (c) for different Cu/Co ratio at 0 V in 100 mM KNO3+ 1 M KOH electrolyte (catalysts loading was 5 mg cm−2).\({{{\mbox{FE}}}}_{{{{\mbox{NH}}}}_{3}}\)(d) and NH3product yield (e) at different electrode potentials on Cu50Co50, pure Cu and pure Co catalysts modified Ni foam (catalysts loading was 5 mg cm−2). Comparison of the electrocatalytic NO3-RR performances of Cu50Co50modified Ni foam with other extensively reported electrocatalysts (f).\({{{\mbox{FE}}}}_{{{{\mbox{NH}}}}_{3}}\)and\({{{\mbox{Yield}}}}_{{{\mbox{mass}}}-{{{\mbox{NH}}}}_{3}}\)on Cu50Co50/Ni foam under the applied potential of −0.2 V during 10 periods of 1 h electrocatalytic NO3-RR (g) (catalysts loading was 5 mg cm−2). The time-dependent concentration of NO3−, NO2−and NH3and corresponding FE over Cu50Co50modified Ni foam at −0.1 V (h) (catalysts loading was 5 mg cm−2). Error bars represent the standard deviations calculated from three independent measurements. When the η reached 590 mV (at 0.1 V), the \({{{{{\rm{FE}}}}}}_{{{{{{\rm{NH}}}}}}_{3}}\) got about 65% on Cu 50 Co 50 (Fig. 3d and Supplementary Fig. S23 ). In comparison, the \({{{{{\rm{FE}}}}}}_{{{{{{\rm{NH}}}}}}_{3}}\) was around 21% on Cu at 0.1 V (Fig. 3d ), with NO 2 − as the main product. As the electrode potential shifted negatively, the intermediate NO 2 − was rapidly reduced (Supplementary Fig. S23 ). At −0.2 V, the \({{{{{\rm{FE}}}}}}_{{{{{{\rm{NH}}}}}}_{3}}\) on Cu 50 Co 50 achieved 100 ± 1%, and \({j}_{{{{{{\rm{NH}}}}}}_{3}}\) reached 1035 mA cm −2 (Supplementary Fig. S24b ), corresponding to an NH 3 production rate of 4.8 mmol cm −2 h −1 that is about two and eight times higher than the ones obtained on monometallic Co and Cu (Fig. 3e and Supplementary Fig. S25 ), respectively. Based on the charge consumed during the CuCo electrodeposition on the Ni foam substrate, the mass activity of NH 3 yield ( \({{{{{\rm{Yield}}}}}}_{{{{{\rm{mass}}}}}-{{{{{\rm{NH}}}}}}_{3}}\) ) on Cu 50 Co 50 was estimated roughly to 960 mmol g cat −1 h −1 at 0.2 V. The obtained \({{{{{\rm{Yield}}}}}}_{{{{{\rm{mass}}}}}-{{{{{\rm{NH}}}}}}_{3}}\) was slightly underestimated since hydrogen evolution was observed during CuCo electrodeposition. It should be noted that the production of NH 3 from electrocatalytic NO 3 − RR is currently at a laboratory scale. More follow-up pilot tests and scale-up work are required to meet the industrial demands. Based on the preliminary calculations, we consider that our work inspired by the bifunctional nature of nitrite reductase, provides a new expectation and shows a great prospect, and after further development could compete with the well-established Haber–Bosch process [12] , [32] which currently shows a \({{{{{\rm{Yield}}}}}}_{{{{{\rm{mass}}}}}-{{{{{\rm{NH}}}}}}_{3}}\) of ca. 200 mmol g cat −1 h −1 at industrial scale. The potential window for \({{{{{\rm{FE}}}}}}_{{{{{{\rm{NH}}}}}}_{3}}\) above 90% was wide and ranged from −0.1 to −0.4 V (Fig. 3d ). Ten cycles of electrolysis at constant potential were performed to check the stability of Cu 50 Co 50 (Fig. 3g ) and the results displayed a stable \({{{{{\rm{FE}}}}}}_{{{{{{\rm{NH}}}}}}_{3}}\) exceeding 90% over the cycles. According to the SEM analysis, the decay of the yield for NH 3 would be due to the nanosheet agglomeration after the consecutive recycling tests (Supplementary Fig. S26a , b). Furthermore, XRD (Supplementary Fig. S26c ) and XPS (Supplementary Fig. S26d , e ) analysis was also performed on the samples after the consecutive recycling tests, and the results demonstrated negligible changes in the chemical compositions and oxidation states, which confirmed the excellent stability of the catalyst. The concentration of NO 3 − in real wastewater can vary from 0.88 mmol L −1 to 1.95 mol L −1 [33] . Therefore, NO 3 − RR on Cu 50 Co 50 was performed at a wide range of NO 3 − concentrations (1–100 mmol L −1 ). The \({{{{{\rm{FE}}}}}}_{{{{{{\rm{NH}}}}}}_{3}}\) was maintained above 95% in the whole range of NO 3 − concentrations (Supplementary Fig. S27 ) at −0.1 V. The NO 3 − RR in neutral conditions was carried out on Cu 50 Co 50 catalysts at −0.2 V in an electrolyte solution of 0.1 M KNO 3 + 0.5 M K 2 SO 4 . The current density of NO 3 − RR on Cu 50 Co 50 in a neutral condition was higher than the one on monometallic Cu and Co, and the \({{{{{\rm{FE}}}}}}_{{{{{{\rm{NH}}}}}}_{3}}\) over Cu 50 Co 50 was more than 90% (Supplementary Fig. S28 ). These experiments demonstrated the excellent property of Cu 50 Co 50 toward NO 3 − recovery in various environmental wastewater systems. In batch conditions with an initial nitrate’s concentration of 100 mmol L −1 ( ca . 6200 ppm) at a reduction potential of −0.1 V and after 10 h, the nitrate’s removal efficiency reached 99.5%, with a \({{{{{\rm{FE}}}}}}_{{{{{{\rm{NH}}}}}}_{3}}\) of 96% (Fig. 3h ). The remaining NO 3 − in the solution was 31 ppm which was much lower than the limitations fixed by the World Health Organization for drinking water, (i.e., 50 ppm) [34] . Several processes can be then considered for further extracting NH 3 , such as air stripping, ion exchange, struvite precipitation, etc. [35] . Electrochemical in situ FTIR, SHINERS and DFT calculations were conducted to elucidate the reaction mechanism as well as the origin of the different activities observed between the catalysts. Electrochemical in situ FTIR analysis of NO 3 − RR The electrochemical thin-layer in situ FTIR can track intermediates in solution within the thin-layer (thickness around 10 μm) between the electrode and IR window and species adsorbed on the electrode surface [36] . A reference spectrum (R Ref ) at reference potential ( E R , 0.4 V) was firstly acquired, and then the potential was stepped to studied potentials ( E S ) and to collect working spectra (R S ). The resulting spectra were represented as relative changes in the reflectance: ΔR/R = (R S -R ref )/R Ref . As a result, the downward band in the resulting spectra indicated the formation of NO 3 − intermediates at E S , while the upward band referred to the consumption of NO 3 − . The FTIR peaks observed on Cu 50 Co 50 , Cu, and Co are compiled in Supplementary Table S3 . As illustrated in Fig. 4 , in the potential range from 0.4 to −0.2 V, the absorption bands were assigned to intermediates present in the electrolyte, since the wavenumbers of all the absorption bands were independent of the working potential [37] . In Fig. 4a , five obvious absorption bands appeared in the infrared spectra of Cu 50 Co 50 viz. (1) At the working potential of 0.2 V, close to the onset potential of the LSV curve, the upward absorption bands at 1392 and 1354 cm −1 were ascribed respectively to N-O symmetric and asymmetric stretching vibration of NO 3 − [38] , indicating consumption of NO 3 − species in the thin layer; (2) at the same time, the downward band at 1236 cm −1 appeared and was attributed to N-O antisymmetric stretching vibration of NO 2 − [39] , indicating NO 2 − formation from NO 3 − reduction; (3) with potential negatively moving to 0.1 V, another intermediate observed around 1110 cm −1 was ascribed to -N-O- stretching vibration of hydroxylamine (NH 2 OH) [39] , [40] , which was a key intermediate for NH 3 formation; (4) The upward band around 1638 cm −1 was attributed to water electrolysis responsible of hydrogen generation involved in the hydrodeoxidation of NO 3 − in the solution of thin-layer [41] . Fig. 4: Electrochemical in situ FTIR spectra. Electrochemical thin-layer in situ FTIR spectra of NO 3 − RR on Cu 50 Co 50 ( a ), Cu ( b ), and Co ( c ) in 100 mM KNO 3 + 1 M KOH. d \(\frac{{{{{{\rm{I}}}}}}_{{{{{{\rm{NO}}}}}}_{2}^{-}}}{{{{{{\rm{I}}}}}}_{{{{{{\rm{NH}}}}}}_{2}{{{{\rm{OH}}}}}}+{{{{{\rm{I}}}}}}_{{{{{{\rm{NO}}}}}}_{2}^{-}}}\) ratio at different electrode pot e ntials. ATR-FTIR spectra on Cu 50 Co 50 ( e ), Cu ( f ), and Co ( g ) in 1 M KOH. Full size image The FTIR spectra collected on Cu (Fig. 4b ) were very similar to the Cu 50 Co 50 catalyst’s ones, indicating that the NO 3 − RR behaviors were similar for both catalysts. However, the NO 3 − consumption on Cu at a potential of 0.1 V was 100 mV more negative than the one obtained on Cu 50 Co 50 , indicating a better kinetic with the latter one. In addition, with the negative shift of the working potential, the band intensity of NO 2 − relative to the sum intensity of NO 2 − and NH 2 OH production (i.e., \(\frac{{{{{{\rm{I}}}}}}_{{{{{{\rm{NO}}}}}}_{2}^{-}}}{{{{{{\rm{I}}}}}}_{{{{{{\rm{NH}}}}}}_{2}{{{{\rm{OH}}}}}}+{{{{{\rm{I}}}}}}_{{{{{{\rm{NO}}}}}}_{2}^{-}}}\) ) on Cu 50 Co 50 dropped down sharply, while the \(\frac{{{{{{\rm{I}}}}}}_{{{{{{\rm{NO}}}}}}_{2}^{-}}}{{{{{{\rm{I}}}}}}_{{{{{{\rm{NH}}}}}}_{2}{{{{\rm{OH}}}}}}+{{{{{\rm{I}}}}}}_{{{{{{\rm{NO}}}}}}_{2}^{-}}}\) ratio was almost independent of the potential on Cu (Fig. 4d ). The two phenomena, i.e., the appearance of NH 2 OH after the formation of NO 2 − and the increase of NH 2 OH at the expense of the consumption of NO 2 − , suggested that *NH 2 OH was obtained by the deep hydrogenation of *NO 2 [42] . The \(\frac{{{{{{\rm{I}}}}}}_{{{{{{\rm{NO}}}}}}_{2}^{-}}}{{{{{{\rm{I}}}}}}_{{{{{{\rm{NH}}}}}}_{2}{{{{\rm{OH}}}}}}+{{{{{\rm{I}}}}}}_{{{{{{\rm{NO}}}}}}_{2}^{-}}}\) ratio on Cu 50 Co 50 was much lower than the one on Cu catalyst, demonstrating that alloying Cu with Co could deeply enhance the hydrogenation of *NO 2 to the final product NH 3 on Cu/Co alloy catalysts. Thereby we speculated that Co sites were responsible for the variation of the \(\frac{{{{{{\rm{I}}}}}}_{{{{{{\rm{NO}}}}}}_{2}^{-}}}{{{{{{\rm{I}}}}}}_{{{{{{\rm{NH}}}}}}_{2}{{{{\rm{OH}}}}}}+{{{{{\rm{I}}}}}}_{{{{{{\rm{NO}}}}}}_{2}^{-}}}\) ratio, owing to their excellent protons’ adsorption (*H) capacity, as it will be demonstrated in the next section, promoting the hydrodeoxidation of *NO 2 to *NH 2 OH according to Eqs. ( 3 ) and ( 4 ): [43] 
    *NO_2+2*H→*NO+H_2O
 (3) 
    *NO+3*H→*NH_2OH
 (4) On pure Co (Fig. 4c ), no spectra bands of NO 3 − RR were detected until the working potential negatively shifted to 0 V. The absence of NO 2 − on the Co catalyst suggested a low NO 2 − accumulation in the thin layer solution, corroborating very well first the results obtained from the K–L equation where the Co catalyst was more inclined to perform continuous hydrogenation of NO 3 − to NH 3 via an 8-electrons transfer and second the lower Tafel slope in the Peak S2 region data. In comparison with thin-layer in situ FTIR, attenuated total reflection in situ FTIR analysis (ATR-FTIR) is more sensitive to the signal of adsorbed species on catalysts’ surfaces [44] . Two weak vibration bands of adsorbed NO in two different adsorption modes (“bridge” and “on top”) were detected at 1557 and 1639 cm −1 on the Cu 50 Co 50 catalyst (Supplementary Fig. S29a ) [38] , [45] . Interestingly, a downward band center at 2109 cm −1 at 0.5 V was observed in NO 3 – free electrolyte on Cu 50 Co 50 (Fig. 4e ), and the band center was negatively shifted to 2085 cm −1 at −0.4 V, yielding a Stark turn rate of 26.7 cm −1 V −1 . These IR features could be attributed to adsorbed *H on the Cu 50 Co 50 surface, and indicated also the enhancement of *H adsorbed on the Cu 50 Co 50 surface at a higher η, which is consistent with the reported studies [46] , [47] . The fact that *H was observed on Cu 50 Co 50 and Co (around 2110 cm −1 ) (Fig. 4e, g and Supplementary Fig. S30c ) while being absent on Cu (Fig. 4f and Supplementary Fig. S30b ), indicated that *H on Cu 50 Co 50 was mainly attributed to water dissociation on Co sites. When the potential negatively shifted, the intensity of Co-H gradually raised, demonstrating that more *H were generated which in turn enhanced the hydrodeoxidation reaction and gave a lower \(\frac{{{{{{\rm{I}}}}}}_{{{{{{\rm{NO}}}}}}_{2}^{-}}}{{{{{{\rm{I}}}}}}_{{{{{{\rm{NH}}}}}}_{2}{{{{\rm{OH}}}}}}+{{{{{\rm{I}}}}}}_{{{{{{\rm{NO}}}}}}_{2}^{-}}}\) ratio value. The wavenumber attributed to *H on Co was slightly higher than the one on Cu 50 Co 50 , indicating a stronger affinity of *H for pure Co catalyst. In the presence of NO 3 − , Co-H was still present in the spectra of pure Co (Supplementary Fig. S30c ), while it was vanished in the spectra of Cu 50 Co 50 (Supplementary Fig. S30a ). This could be explained by the fact that *H could adsorb quickly on Co sites inhibiting the adsorption of NO x, then the adsorbed hydrogen can react with the equivalent amount of *NO x on nearby Cu sites giving a high reaction kinetics. In the case of monometallic Co, the active sites are majorly occupied by *H species preventing the adsorption of NO x onto the catalyst’s surface, leading to weak activity. The presence of active hydrogen (H*) in the reaction process was also verified by electron paramagnetic resonance (EPR) analysis on Cu 50 Co 50 catalyst (Supplementary Fig. S31 ) using 5,5-dimethyl-1-pyrroline N -oxide (DMPO) as a spin trap [48] . The intensity of the EPR signal of the DMPO-H adduct on the Cu 50 Co 50 catalyst decreased when nitrate was added into the electrolyte, indicating the consumption of active hydrogen during NO 3 − RR. These results were consistent with the ATR-FTIR analysis. Based on the coupling of thin-layer in situ FTIR and ATR-FTIR analysis, therefore, we proposed the following pathway for the NO 3 − RR on Cu 50 Co 50 : NO 3 − → *NO 3 → *NO 2 → *NH 2 OH → *NH 3 , where *H on Co sites can promote the deep hydrodeoxidation of NO 2 − to NH 2 OH. SHINERS analysis of NO 3 − RR The reaction intermediates provided by electrochemical in situ FTIR spectra were still insufficient to figure out the overall roadmap of NO 3 − RR to NH 3 , in this aim, SHINERS spectra of the catalysts were collected to probe the catalysts’ surface during the reaction. Supplementary Table S4 compiled the Raman scattering peaks observed during NO 3 − reduction on Cu 50 Co 50 , Cu, and Co, which were not detected on Au@SiO 2 (Supplementary Fig. S32 ). The wavenumber below 750 cm −1 corresponds mainly to the chemical properties of the catalyst’s surface [43] . SHINERS spectra of Cu 50 Co 50 , Cu, and Co, in this section, were summarized and shown in Fig. 5 . At 0.6 V, a characteristic band at 625 cm -1 associated with Cu 2 O [49] was observed on Cu and Cu 50 Co 50 (Fig. 5a, b ), indicating partial oxidation of the catalysts surface due to air exposition before NO 3 − RR; these results were consistent with the XPS data. As the working potential decreased to 0.3 V, the band intensity of Cu 2 O gradually shrank, and a peak at 714 cm −1 emerged in replacement and was associated with the bending mode of free Cu-OH ad [50] , [51] , indicating a gradual reduction of Cu before NO 3 − RR started to occur at 0.2 V. Besides, the band at 431 cm −1 can be assigned to Cu-O x due to the adsorption of oxynitride on Cu surface [51] , and the band’s intensity increased as the potential moved negatively. For Co (Fig. 5c ), a band at 568 cm −1 was also observed, associated with the formation of Co-O x caused by the same oxynitride species adsorbed on the catalyst’s surface [52] . Fig. 5: Electrochemical SHINERS spectra of NO 3 − RR. SHINERS spectra between 230–750 cm −1 on Cu 50 Co 50 ( a ), Cu ( b ), and Co ( c ). SHINERS spectra between 750–1700 cm −1 on Cu 50 Co 50 ( d ) in 100 mM KNO 3 + 10 mM KOH during cathodic polarization from 0.7 to −0.1 V. Full size image In addition, the signals of NO 3 − and its reduced intermediates adsorbed on the catalysts’ surface were observed in the spectra between 750 and 1700 cm −1 . As the potential decreased from 0.7 to −0.1 V, several peaks appeared in sequences on Cu 50 Co 50 (Fig. 5d ) viz. (1) At open circuit potential (OCP) and 0.7 V, the only obvious peak viewed at around 1049 cm −1 was attributed to the symmetric NO 3 − stretching from solution NO 3 − species [53] . (2) When the potential was decreased to 0.4 V, the NO 3 − species in the solution started to adsorb on the surface of Cu 50 Co 50 since four peaks appeared in three different forms as NO stretching vibration from the unidentate nitrate near 998 cm −1 , symmetric and antisymmetric stretching vibration of the NO 2 group from the chelated nitro configuration around 1125 and 1254 cm −1 [54] , and the N=O stretching vibration of the bridged nitro group closed to 1439 cm −1 , respectively [55] . (3) As the working potential shifted negatively further to 0.2 V, the symmetric NO 3 − stretch of *NO 3 − appeared around 1028 cm −1 [56] , [57] and symmetric bending vibrations of the HNH near 1315 and 1374 cm −1 were apparent; [55] , [57] N=O stretch of HNO [56] was visible around 1540 cm −1 . (4) When the potential negatively shifted further to 0.1 V, the HNO peak near 1540 cm −1 disappeared quickly; meanwhile, the antisymmetric bending vibration of the HNH of NH 3 at 1591 cm −1 came out [58] , which indicated an efficient formation of NH 3 from HNO hydrodeoxidation. The SHINERS spectra on Cu and Co catalysts (Supplementary Fig. S33a, b ) were similar to the one of Cu 50 Co 50 , but a new peak close to 800 cm −1 related to the bending vibration of NO 2 − group was only observed on Cu (Supplementary Fig. S33a ) [26] . This could be due to the accumulation of NO 2 − species near by the Cu surface due to its poor ability for deep NO 2 − hydrodeoxidation properties. The intensity of \({\nu }_{{{{{{\rm{s}}}}}}({{{{{\rm{N}}}}}}{O}_{3}^{-})}\) from NO 3 − species in solution on Co at low overpotential was similar to the one on Cu 50 Co 50 and Cu, however, the band’s intensities of all the intermediates formed on Co were very weak (Supplementary Fig. S33b ), meaning that a low amount of *NO 3 − species and its derivates were adsorbed on the Co surface. It can be rationally speculated that the affinity of *H species to the Co surface was such strong that the active sites on the Co catalyst were majorly occupied by *H species leading to low coverage of *NO 3 − species, bringing a \({{{{{\rm{FE}}}}}}_{{{{{{\rm{NH}}}}}}_{3}}\) close to 85% (Fig. 3b ) at the expense of a low current density of NO 3 − RR of 25.4 mA cm −2 (Supplementary Fig. S24a ) at 0 V. Similarly, *H species affinity for Cu surface was so weak that most active sites were occupied by *NO 3 − species, leading to a relatively high current density up to 104.8 mA cm −2 (Supplementary Fig. S24a ) and yet an unsatisfactory \({{{{{\rm{FE}}}}}}_{{{{{{\rm{NH}}}}}}_{3}}\) of 32% (Fig. 3b ). Therefore only if a balanced coverage of *H and *NO 3 species is achieved, a satisfactory \({{{{{\rm{FE}}}}}}_{{{{{{\rm{NH}}}}}}_{3}}\) and j can be simultaneously obtained, which is the case with Cu 50 Co 50 where \({{{{{\rm{FE}}}}}}_{{{{{{\rm{NH}}}}}}_{3}}\) and j were 88% 394.6 mV respectively. With combined electrochemical in situ FTIR and SHINERS spectroscopic analysis, the NO 3 − RR pathway on Cu, Co and CuCo was proposed as a series of deoxygenation reactions according to the following path, NO 3 − → *NO 3 → *NO 2 → *NO, accompanied by a series of hydrogenation reactions: *NO → *NOH → *NH 2 OH → * NH 3 → NH 3 . DFT calculations Based on all the aforementioned observations and to shed light on the NO 3 − RR mechanism on Cu, Co, and CuCo at the atomic level, the density functional theory (DFT) calculations were conducted and the Gibbs free energies (ΔG) of *NO 3 species and their derivates on Cu(111), Co(111) and CuCo(111) surface were presented in Fig. 6a . Fig. 6: DFT calculations of NO 3 − RR and HER on Cu(111), Co(111), and CuCo(111). Reaction-free energies for different intermediates of NO 3 - RR ( a ) and HER ( b ) at −0.2 V vs. RHE on CuCo(111), pure Cu(111), and pure Co(111) surface, respectively. Full size image In terms of thermodynamics, the rate-determining step (RDS) on Cu(111), Co(111) and CuCo(111) was the initial *NO 3 adsorption step and lower energy was required on CuCo(111) (0.17 eV), compared to Cu(111) (0.61 eV) and Co(111) (0.34 eV), indicating stronger adsorption of NO 3 − species on CuCo(111) [15] , [59] . Interestingly, the ΔG of the initial *NO 3 species on Co(111) was lower than the one obtained on Cu(111), which should lead to better NO 3 − RR performances. However, this result contradicted the fact that \({\eta }_{{@10{{{{{\rm{mA}}}}}}{{{{{\rm{cm}}}}}}}^{-2}}\) of NO 3 − RR on Cu was 503 mV more positive than on Co ( \({\eta }_{{@10{{{{{\rm{mA}}}}}}{{{{{\rm{cm}}}}}}}^{-2}}\) of 690 mV). This inconformity could be explained by a strong competition of *H species on the catalyst sites’ surface compared to nitrogenous species, as proved by in situ FTIR and SHINERS analysis. Indeed, Co was capable of promoting hydrogenation during the NO 3 − RR by transferring in situ *H species [13] , because of its excellent adsorption for *H species [60] . However, the excessive adsorption of *H can reduce the coverage of *NO 3 species and their intermediates, thereby weakening the electrochemical activity toward NO 3 − RR. Compared with the ΔG of *NO 3 and *H on Co(111) (Fig. 6b and Supplementary Table S11 ), the adsorption for *H was stronger, but the adsorption for NO 3 − was poor. With the incorporation of the Cu atom, the electronic structure changed, enhancing the adsorption of NO 3 − species on CuCo(111) and furthermore, the partial replacement of Co sites with Cu sites also reduced the coverage of *H species. Based on the comprehension of the results discussed above, the redistribution of electrons in Cu 50 Co 50 facilitated the electrons transfer rate and uplifted the catalytic kinetic of the NO 3 − RR (Supplementary Figs. S6 , S7 ). The fair coverage of *H and *NO 3 species were important to obtain simultaneously a high \({{{{{\rm{FE}}}}}}_{{{{{{\rm{NH}}}}}}_{3}}\) and \({j}_{{{{{{\rm{NH}}}}}}_{3}}\) . Co-adjustment of Cu and Co sites on Cu 50 Co 50 can balance the adsorption energy between *H and *NO 3 species, not only by lowering the energy barrier of NO 3 − reduction but also by improving the hydrogenation capability with the enhanced *H adsorption compared with pure Cu, and at the same time avoiding the excessive *H occupation of the active sites compared to pure Co. To conclude, we presented a novel Cu-based catalyst able to mimic the Cu core center of the Cu-NIR for the electrocatalytic NO 3 − reduction. The addition of Co to Cu formed a micro-pine structure with nanosheets and enhanced dramatically the proton availability over the surface of the catalyst from water electrolysis, resulting in an almost full Faraday efficiency of NH 3 production at an ampere-level current density of 1035 mA cm −2 at −0.2 V. This process exhibited a high activity and could be proposed as a sustainable and eco-friendly complementary route of NH 3 production. In batch conditions, the catalyst was able to achieve a \({{{{{\rm{FE}}}}}}_{{{{{{\rm{NH}}}}}}_{3}}\) of 96% and a nitrate’s removal of 99.5%, from an initial concentration of 6,200 ppm, reaching a final concentration of 31 ppm after 10 h of reaction, lower than the limitations fixed by the World Health Organization for drinking water. A mechanism was established by combining in situ FTIR and SHINERS spectroscopic investigations and DFT calculations. The synergy between Cu and Co can reduce the high energy barrier of the rate-determining step of the initial *NO 3 adsorption step on Cu, due to a regulation of the electronic structure. The ΔG of the hydrogenation of the intermediate species, *NO x , could also be reduced due to the facile adsorption of *H species on Co(111) compared to Cu(111). We proposed that a rational control of the *H adsorption over the surface of the bimetallic catalyst is the key to managing further adsorption of intermediates from NO 3 − RR to achieve excellent performances. This discovery can provide an additional dimension to research into surface adsorption-modulated bimetallic catalysts for highly reactive hydrodeoxidation reactions and can provide a novel strategy for the development of multi-component heterogeneous catalysts for efficient NH 3 production and wastewater treatment. Preparation of Cu x Co y , Cu, and Co catalysts The catalysts were prepared via an electrodeposition process under the current density of 50 mA cm −2 for 300 s in a two-electrodes system where a platinum plate was used as the counter electrode and the Ni foam as the working electrode. Ni foams were pretreated with acetone and ethanol, and then repeatedly rinsed with ultrapure water and dried under a heating lamp. The deposition electrolyte (50 mL) comprised of 0.015 M trisodium citrate pentahydrate solutions and 50 mM CuSO 4 + CoSO 4 [61] , [62] . The Cu x Co y catalysts with Cu:Co ratios of 65:35, 50:50, and 15:85, denoted as Cu 65 Co 35 , Cu 50 Co 50 , and Cu 15 Co 85 , were obtained in the deposition solutions with the ratio of CuSO 4 to CoSO 4 as 60:40, 45:55, and 10:90, respectively. The Cu and Co catalysts were prepared. The preparation for pure Cu and Co catalysts followed the same steps as the Cu x Co y synthesis, except that only CuSO 4 or CoSO 4 solution was present in the electroplating solution. The catalysts were finally rinsed with ultrapure water and dried under the protection of Ar. Material characterization Morphology and elemental composition were characterized using a scanning electron microscope (SEM, ZEISS Sigma) with an energy dispersive X-ray spectrometer at an operating voltage of 15 kV. The lattice arrangement was observed using a high-resolution transmission electron microscope (HRTEM, FEI-Tecnai G2 F20) at an accelerated voltage of 200 kV. The chemical composition was analyzed by an inductively coupled plasma emission spectrometer (ICP-OES, Thermo Fisher iCap 7000). X-ray diffractometer (XRD, SmartLab-SE) with Cu-Kα X-ray source was used for crystal material structure analysis. Al Ka X-ray excited Thermo Fisher Scientific Nexsa X-ray Photoelectron spectrometer (XPS, Nexsa) was used for chemical state analysis. All XPS spectra were corrected with a C 1 s spectral line of 284.8 eV. X-ray absorption fine structure (XAFS) spectra at Cu K-edge and Co K-edge were obtained on the 1W1B beamline of Beijing Synchrotron Radiation Facility (BSRF) operated at 2.5 GeV and 250 mA. Standard data processing, including energy calibration and spectral normalization of the raw spectra was performed using Athena software. Electrochemical test The electrochemical measurements were performed using a three-electrodes system connected to the CHI 760E workstation (Chenhua, Shanghai) in a homemade H-type cell (separated by Nafion 117 membrane; with magnetic stirring of 1000 rpm). The Nafion 117 was preprocessed according to the reported procedures. The Cu x Co y /Ni foams (0.5 cm 2 × 0.5 cm 2 ) were used as working electrodes, and platinum plate and Hg/HgO electrode (filled with 1 M KOH solution) were used as counter and reference electrodes, respectively. Before the testing, all the catalysts were electro-reduced at −0.2 V vs . RHE for 600 s in 1 M KOH solution to eliminate surface oxidation. 1 M KOH aqueous solution containing different KNO 3 − concentrations (5, 10, 50, and 100 mM) were used as an electrolyte (30 ml). The electrolyte was bubbled with Ar to remove O 2 and N 2 for 10 min before the experiment. The electrochemical linear voltammetry (LSV) curves were obtained in a single cell. The current density was normalized to the geometric electrode area (0.25 cm 2 ) unless otherwise specified. The cyclic voltammetry curves in electrochemical double-layer capacitance (C dl ) determination were measured in a potential window where no Faradaic process occurred in an electrolyte of 1 M KOH at different scanning rates of 20, 40, 60, 80, and 100 mV s −1 . All the potentials were converted to the RHE reference scale by E (V vs . RHE) = E (V vs. Hg/HgO) + 0.0591 × pH + 0.098. Note that NH 3 volatilization in the 1 M KOH electrolytes (pH 13.6) is negligible during the 1-h electrolysis. Kinetic evaluation The electrochemical kinetic analysis of NO 3 − RR was performed based on the Koutecký–Levich (K–L) equation, as shown in Eq. ( 5 ): 
    1/i_m=1/i_K+1/0.2nFD^2/3ν^-1/6Cω^1/2
 (5) Where i m is the test current; i K is the kinetic current of NO 3 − reduction; n is the number of electrons transferred in the reaction; F is the Faraday constant, 96485 C mol −1 ; D represents the effective diffusion coefficient of 0.1 mol L −1 NO 3 − at 25 °C, 1.4 × 10 −5 cm 2 s −1 ; υ represents the kinematic viscosity of water at 25 °C, 1 × 10 −6 m 2 s −1 ; C is NO 3 − concentration, mmol L −1 ； ω is the electrode speed, rpm. The working electrode was prepared as follows: (1) 5 mg of catalyst powder dropped down from Cu x Co y /Ni foam and was dispersed in the solution of 600 μL isopropanol + 380 μL ultrapure water + 20 μL 5% Nafion solution, and then sonicated for at least 1 h to get a homogeneous ink; (2) 10 μL ink was drop-casted onto the rotating disk electrode (Ø, 0.196 cm2) with the loading of 0.255 mg catalyst cm −2 for the further LSV analysis at different speeds (100, 225, 400, and 625 rpm) with a scan rate of 10 mV s −1 . A platinum electrode and an Hg/HgO electrode were used as counter electrode and reference electrode, respectively. An aqueous solution of 1 mol L −1 KOH containing 100 mmol L −1 KNO 3 was used as the electrolyte. Ar was used to purge the dissolved O 2 and N 2 from the electrolyte. Product detection and efficiency calculation The NH 3 concentration was quantified by the Nessler Reagent method [28] . The electrolytes sampled after electrolysis for 1 h were first neutralized with 0.5 M H 2 SO 4 and then mixed with 6.25 mL ultrapure water and 0.25 mL of Nessler reagent for the chromogenic reaction. The absorbance of the mixed solution was measured at a wavelength of 420 nm after keeping it at room temperature for 30 min. The quantitation of NH 3 was performed by the standard curves, which was built using standard NH 4 Cl solutions in 1 M KOH. The 1 H NMR (500 MHz) determination [31] was also carried out to quantify the 14 NH 4 + and 15 NH 4 + after electrolysis at −0.2 V vs . 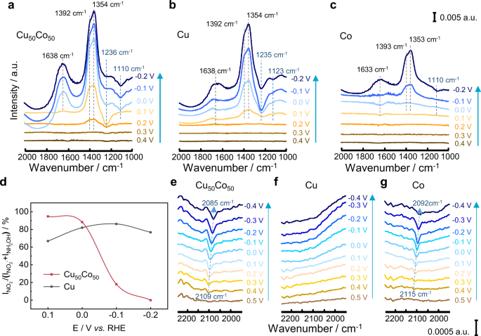Fig. 4: Electrochemical in situ FTIR spectra. Electrochemical thin-layer in situ FTIR spectra of NO3−RR on Cu50Co50(a), Cu (b), and Co (c) in 100 mM KNO3+ 1 M KOH.d\(\frac{{{{{{\rm{I}}}}}}_{{{{{{\rm{NO}}}}}}_{2}^{-}}}{{{{{{\rm{I}}}}}}_{{{{{{\rm{NH}}}}}}_{2}{{{{\rm{OH}}}}}}+{{{{{\rm{I}}}}}}_{{{{{{\rm{NO}}}}}}_{2}^{-}}}\)ratio at different electrode potentials. ATR-FTIR spectra on Cu50Co50(e), Cu (f), and Co (g) in 1 M KOH. RHE for 1 h. The electrolytes were mixed with 0.4 M H 2 SO 4 at a ratio of 500:125 to ensure adequate protonation of NH 3 . Then, 125 μl of the diluted electrolytes or standard solution were mixed with 125 μl of 10 mM maleic acid in DMSO-D6, 50 μl of 4 M H 2 SO 4 , and 300 μl of H 2 O. The NO 3 − and NO 2 − in the solution were quantitatively determined by ion chromatography (IC). The possible gas products of NO 3 − RR, such as H 2 , N 2 , NO, NO 2 , N 2 O, and NH 3 (g) were analysed using a gas chromatography (GC) and online electrochemical mass spectrometry (OEMS) [30] . The Faradaic efficiency was calculated according to the following equation: 
    FE=ncV_catholyteF/Q× 100%
 (6) where c represents the concentration of the product, mol cm -3 ; V catholyte is the volume of catholyte, mL; Q is the total amount of charge consumed, C. The yield rate of NH 3 was calculated according to the following equations: 
    Yield_NH_3=cV_catholyte/St
 (7) 
    Yield_mass-NH_3=cV_catholyte/mt
 (8) where S is the area of the geometrical cathode, cm -2 ; m is the mass of the catalyst on the cathode; t is the time of the electrolysis. Electrochemical in situ FTIR reflection analysis Electrochemical in situ FTIR reflection spectroscopy [44] . Electrochemical thin-layer in situ FTIR spectroscopy measurements were performed on a Nicolet Nexus 8700 FTIR spectrometer equipped with a liquid N 2 -cooled system and MCT-A detector. The glassy carbon electrode loading with catalysts was used as the working electrode, which was pressed vertically on the CaF 2 window plate to form a thin liquid layer with a thickness of about 10 μm. A platinum foil and an Hg/HgO electrode (filled with 1 M KOH solution) were used as the counter electrode and reference electrode, respectively. The incoming infrared beam was approximately aligned with the normal electrode surface. Unless otherwise noted, the sample spectra were averaged from 200 interference spectra with a resolution of 8 cm −1 . Reference spectrum (R Ref ) were collected at 0.4 V, and sample spectra (R S ) were collected in the potential region from 0.4 V to −0.2 V and stepped by 100 mV. The spectra were reported as ΔR/R = (R S − R Ref )/ R Ref . Attenuated Total Reflection in situ FTIR reflection spectroscopy [36] . The gold-plated Si prism with catalysts were assembled into a homemade spectral-electrochemical cell, which contained a carbon sheet as a counter electrode and Hg/HgO electrode as a reference electrode. It was then fixed in a homemade optics system built in the chamber of a Nicolet Nexus 8700 FTIR spectrometer for electrochemical ATR-FTIR measurements at an incidence angle of ca . 65°. The ATR-FTIR spectra were reported in the same way of thin-layer in situ FTIR, except that R Ref was taken at 0.5 V and R S were collected in the potential region from 0.5 to −0.4 V. SHINERS analysis SHINERS spectra were recorded in a custom-made in situ Raman spectroelectrolysis cell using an XplorA confocal microprobe Raman spectrometer (HORIBA Jobin Yvon) [63] . 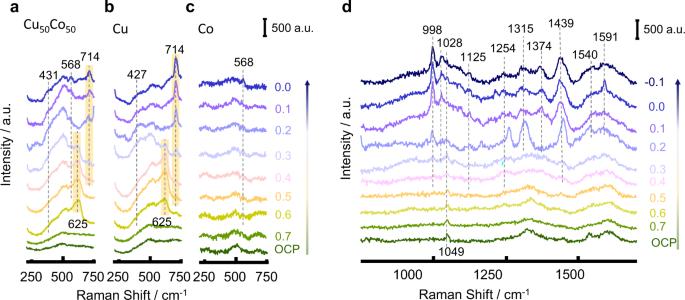Fig. 5: Electrochemical SHINERS spectra of NO3−RR. SHINERS spectra between 230–750 cm−1on Cu50Co50(a), Cu (b), and Co (c). SHINERS spectra between 750–1700 cm−1on Cu50Co50(d) in 100 mM KNO3+ 10 mM KOH during cathodic polarization from 0.7 to −0.1 V. 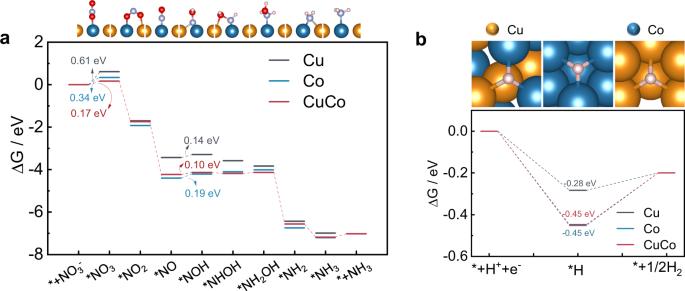Fig. 6: DFT calculations of NO3−RR and HER on Cu(111), Co(111), and CuCo(111). Reaction-free energies for different intermediates of NO3-RR (a) and HER (b) at −0.2 Vvs.RHE on CuCo(111), pure Cu(111), and pure Co(111) surface, respectively. The excitation wavelength of the laser was 637.8 nm and came from a He-Ne laser with a power of about 6 mW. The electrochemically polished gold electrode (diameter 3 mm) was modified by 10 μL catalyst ink with 10 μL homemade shell-isolated gold nanoparticle, which was provided by Prof. Jian-Feng Li at Xiamen University, China, and applied as the working electrode. Hg/HgO electrode was used as the reference electrode, and platinum wires was used as the counter electrode. A long-focus objective (8 mm) of A × 50 magnification was used. A Si wafer (520.6 cm −1 ) was used to calibrate the Raman frequency before the experiment. The SHINERS spectra were obtained using the cumulative results of four tests for 30 s each. EPR Experiments 5,5-dimethyl-1-pyrroline N -oxide (DMPO) was used to capture the instable hydrogen radical to form the DMPO-H adduct to generate EPR spectra [64] . In the experiments, 5 ml electrolyte was mixed with 10 μL DMPO and was deoxygenated by bubbling Ar. The potentiostatic electrolysis was carried out for 5 min in the H-type cell under the protection of Ar. EPR measurement was performed by Bruker EMX-10/12 spectrometer operating at a frequency near 9.5 GHz, sweep width of 200 G and power of 20 mW. DFT calculations All DFT calculations in this work were carried out with the Vienna Ab initio Simulation Package (VASP) [65] . And the projector augmented-wave (PAW) pseudopotential was selected to deal with the core-valence interaction [66] . The generalized gradient approximation (GGA) of Perdew–Burke–Ernzerhof (PBE) was used to account for the exchange and correlation of electronics and the cut-off energy of plane-wave was 600 eV [67] . The energy convergence criterion was within 10 -5 eV and the Hellmann–Feynman force was smaller than 0.01 eV Å −1 on each atom. The converged unit cell models of Cu (3.64 × 3.64 × 3.64 Å 3 ), Co (3.52 × 3.52 × 3.52 Å 3 ), and CuCo (3.78 × 3.49 × 3.49 Å 3 ) were used in DFT calculations, respectively. The dimension of a 2 × 2 supercell of Cu (111) (8.91 × 10.28 Å 2 ), a 2 × 2 supercell of Co (111) (8.62 × 9.95 Å 2 ) and a 2 × 2 supercell of CuCo (111) (9.03 × 9.87 Å 2 ) were used, respectively. These supercells were constructed and contained three layers and a sufficient vacuum layer of 15 Å thicknesses. For the structural optimization, the bottom two layers were fixed and the top layer was fully relaxed [68] . For unit cell geometry optimization, an 8 × 8 × 8 k-point analysis was used. A grid of 3 × 3 × 1 k-point mesh was used for these supercell calculations [15] . The calculations of all molecules and intermediate species on Co(111) and CuCo(111) were performed with spin polarization [69] . Dipole corrections in the z direction were included in all computations to minimize inaccuracies in the total energy because of simulated slab interactions. The spin polarization was not taken into account in the calculations of intermediate species on Cu(111) due to the spin polarization did not affect the Cu (111) calculations.